High internal quantum efficiency in fullerene solar cells based on crosslinked polymer donor networks The power conversion efficiency of organic photovoltaic cells depends crucially on the morphology of their donor–acceptor heterostructure. Although tremendous progress has been made to develop new materials that better cover the solar spectrum, this heterostructure is still formed by a primitive spontaneous demixing that is rather sensitive to processing and hence difficult to realize consistently over large areas. Here we report that the desired interpenetrating heterostructure with built-in phase contiguity can be fabricated by acceptor doping into a lightly crosslinked polymer donor network. The resultant nanotemplated network is highly reproducible and resilient to phase coarsening. For the regioregular poly(3-hexylthiophene):phenyl-C 61 -butyrate methyl ester donor–acceptor model system, we obtained 20% improvement in power conversion efficiency over conventional demixed biblend devices. We reached very high internal quantum efficiencies of up to 0.9 electron per photon at zero bias, over an unprecedentedly wide composition space. Detailed analysis of the power conversion, power absorbed and internal quantum efficiency landscapes reveals the separate contributions of optical interference and donor–acceptor morphology effects. The power conversion efficiency (PCE) of donor–acceptor (DA) photovoltaic (PV) cells depends on the spectral absorption and the bias-dependent internal quantum efficiency of the cell [1] , [2] . To achieve a high internal quantum efficiency, the heterostructure needs to have the appropriate interface electronic structure combined with the appropriate morphology to give efficient exciton dissociation and transport of the charge carriers to the collection electrodes without recombination. The ideal morphology is widely believed to comprise donor and acceptor phases intimately mixed at the exciton diffusion length scale (~10 nm), but contiguously extended over the much larger photoactive layer thickness (100–250 nm). These two conflicting requirements however present a formidable challenge that has not yet been possible to address by design. In addition, there is a further challenge that the morphology needs to be stable and reliably manufacturable over large areas. Although the standard approach of spontaneous DA demixing [3] in films under thermal [4] or solvent vapour [5] annealing conditions, or in the presence of solvent additives [6] , can provide, in some cases, a suitable ultrafine morphology, such as in the poly(3-hexylthiophene):phenyl-C 61 -butyrate methyl ester (P3HT:PCBM) DA system, the morphology still cannot presently be predefined. Furthermore, the processing window is rather narrow and variable [4] , [5] , [6] , [7] , [8] , [9] , with the desired morphology itself being metastable [10] , [11] , [12] , [13] , [14] and prone to over-coarsening that degrades cell performance. We report here that by infiltrating or doping the molecular acceptor into a lightly crosslinked polymer donor network, the ideal interpenetrating DA heterostructure can be closely approached. This provides remarkably high internal quantum efficiencies to the solar cells with consistency across a wide composition space. The morphology produced is robust to further coarsening, and to film-processing conditions. We demonstrate this on the P3HT:PCBM system, and show that a further improvement in device performance can be obtained over the relatively high internal quantum efficiencies that are already reached in the usual demixed biblend films. This improvement is traced to a more optimal morphology in the networks. To crosslink the films, we used a recently developed steric-substituted bis(fluorinated phenyl azide; s -FPA) methodology [15] , [16] . Its key advantage is the non-specificity that allows a wide variety of semiconductor polymers to be crosslinked at a sufficiently low crosslinker concentration that does not degrade their crucial semiconductor properties. We have previously demonstrated this provides viable new heterostructures for light-emitting diodes, field-effect transistors and PV cells [16] . The work here demonstrates the finesse in DA morphology control that can be achieved using polymer networks. A P3HT film is first lightly crosslinked just above its gel point and back-infiltrated with PCBM to the desired volume fraction, whereupon the PCBM nanotemplates the P3HT network to give the ultrafine contiguous DA heterostructure. The low crosslink density plays a crucial role to stabilize the network and frustrate phase coarsening by suppressing long-range diffusion of the polymer chains, but without hindering their local ordering required for high carrier mobility. Since the DA morphology is defined by molecular nanotemplating of the crosslinked network, rather than spontaneous demixing of two ‘free’ components, it is markedly less sensitive to film thickness and processing conditions. This opens a possibility to predefine morphology separately from electronic structure and film thickness, which facilitates the systematic optimization of PV cells and elucidation of their device physics. We illustrate this by performing detailed mapping of the PCE, power absorption and internal quantum efficiency landscapes of these cells. Fabrication of crosslinked P3HT network: PCBM films P3HT films were spin-cast with three weight-to-weight (w/w) % of the s -FPA photocrosslinker ethylene bis(4-azido-2,3,5-trifluoro-6-isopropylbenzoate) [16] onto the intended substrates (for chemical structures, see inset of Fig. 1a ). The films were then exposed to 254-nm deep ultraviolet (DUV) in an N 2 glove box to activate an efficient nitrene-mediated photo crosslinking through the alkyl side chains of P3HT [16] . 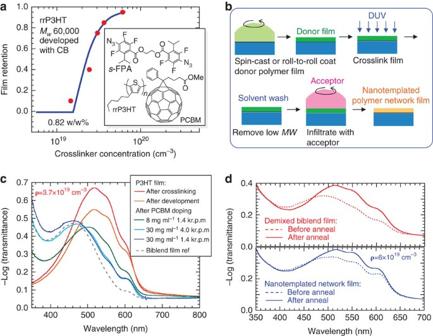Figure 1: Nanotemplating polymer networks. (a) Film-retention characteristics of P3HT usings-FPA as photocrosslinker. Inset gives the chemical structures. (b) Processing schematic. (c) Electronic spectra of key stages: after crosslinking P3HT (dP3HT=77 nm; red), after CB development (65 nm; orange), after PCBM doping at 8 mg ml−1by spin-casting at 1.4k r.p.m. (dPCBM=30 nm; green), or 30 mg ml−1at 4.0k r.p.m. (50 nm; light-blue), or 30 mg ml−1at 1.4k r.p.m. (70 nm; dark-blue); biblend film with (dP3HT,dPCBM)=(55 nm, 45 nm) as reference. Density P3HT, 1.1 g cm−3; PCBM, 1.7 g cm−3. (d) Electronic spectra before and after annealling (140 °C, 10 min; hotplate): demixed biblend film (top) and nanotemplated polymer network film (bottom) withdPCBM/dP3HT~0.7. Figure 1a shows the film-retention characteristics plotted against the s -FPA concentration. These characteristics were measured after solvent washing (often called ‘development’ in the photolithography literature) with chlorobenzene (CB) to remove the uncrosslinked and low-molecular-weight (MW) fractions. As s -FPA exhibits a near-unity crosslinking efficiency [16] , the crosslink density ρ in the film closely follows the crosslinker concentration. The plot shows that film retention occurs above a critical threshold, called the gel point, where an infinite polymer network first emerges (here, ρ ≈2 × 10 19 cm −3 ). The film retention increases towards unity with increasing ρ . Hence network stiffness and porosity can be tuned by ρ . In this work, we set ρ ≈4–6 × 10 19 cm −3 to stay in the lightly crosslinked regime, with roughly one crosslink per 35–50 polymer repeat units. Figure 1: Nanotemplating polymer networks. ( a ) Film-retention characteristics of P3HT using s -FPA as photocrosslinker. Inset gives the chemical structures. ( b ) Processing schematic. ( c ) Electronic spectra of key stages: after crosslinking P3HT ( d P3HT =77 nm; red), after CB development (65 nm; orange), after PCBM doping at 8 mg ml −1 by spin-casting at 1.4k r.p.m. ( d PCBM =30 nm; green), or 30 mg ml −1 at 4.0k r.p.m. (50 nm; light-blue), or 30 mg ml −1 at 1.4k r.p.m. (70 nm; dark-blue); biblend film with ( d P3HT , d PCBM )=(55 nm, 45 nm) as reference. Density P3HT, 1.1 g cm −3 ; PCBM, 1.7 g cm −3 . ( d ) Electronic spectra before and after annealling (140 °C, 10 min; hotplate): demixed biblend film (top) and nanotemplated polymer network film (bottom) with d PCBM / d P3HT ~0.7. Full size image Figure 1b shows a schematic of the film-processing steps. The P3HT donor film is crosslinked and developed with CB as described above. The PCBM acceptor is then doped into this polymer network by spinning from solution. Figure 1c shows the evolution of molecular order in the P3HT network probed by electronic spectroscopy. The electronic spectrum of the crosslinked P3HT film ( ρ =3.7 × 10 19 cm −3 ; red spectrum) is identical to the uncrosslinked one. Thus, its electronic structure is not perceptibly altered by the crosslinks. When this film is washed with CB, it loses 20% of its absorbance (orange spectrum), primarily because of extraction of the low MW fraction. The spectrum of this 65-nm-thick polymer film shows electronic features that are substantially unchanged in relative intensities at 517, 560 and 610 nm, corresponding to the 0→2, 0→1 and 0→0 vibronic transitions [17] . Hence, the retained film exhibits similar molecular order as the initial spin-cast film. When a PCBM solution (8 mg ml −1 in CB) is spun over this film, an amount equivalent to a 30-nm-thick film of PCBM is doped into the P3HT matrix. The polymer absorption diminishes and blue shifts, while the PCBM absorption emerges with onset at 450 nm (green spectrum) [4] . The blue shift arises from (i) disordering of a fraction of the P3HT segments owing to acceptor incorporation and (ii) redistribution of chain segments from in-plane to out-of-plane orientations. The film composition is established using the calibrated absorptivities of P3HT and PCBM, together with the measured initial and final film thicknesses. This is denoted by ( d P3HT , d PCBM ), where d P3HT and d PCBM are, respectively, the effective P3HT and PCBM thicknesses in the film, with total film thickness d given by d P3HT + d PCBM . Some of these compositions have been verified using X-ray photoelectron spectroscopy. This doping is fully reversible, as contact with the pure solvent removes the PCBM and restores the original polymer spectrum. The extent of PCBM doping can be controlled at will through its solution concentration (and spin speed). For example, Fig. 1c also shows the same P3HT film ( d P3HT =65 nm) doped with increasing amounts of PCBM up to 50 vol% ( d PCBM =50 nm, light-blue; 70 nm, dark-blue spectra). In roll-to-roll processing, this could be achieved by film immersion into the requisite bath. Remarkably, a fraction of highly ordered P3HT segments persists in the doped P3HT network even at the highest PCBM volume fraction. This is shown by retention of the ordered 0→0 transition. This is attributed to a molecular ‘scaffolding’ effect. For comparison, the as-cast biblend film exhibits considerably less order at the same PCBM volume fraction (grey dashed spectrum). A subsequent heat treatment at 140 °C promotes further P3HT ordering in both the demixed biblend film [4] , [9] and the crosslinked network film, though the latter still generally achieves better order ( Fig. 1d ). This can be tuned by the crosslink density of the network ( Supplementary Fig. S1 and Supplementary Discussion ). We expect that better order can give the higher carrier mobility needed for more efficient carrier dissociation and higher PV fill factors [10] , [18] . Recent calculations suggest that the mobilities of both electrons and holes need to be larger than ca . 10 −3 cm 2 V −1 s −1 in 220-nm-thick devices to mitigate the space-charge voltage penalty at 1 sun (unpublished results). The PCBM promotes an isotropic orientation of the P3HT network that should facilitate hole transport in the film-thickness direction [19] . High-resolution imaging of the nanotemplated polymer network To characterize the P3HT morphology, we performed high-resolution transmission electron microscopy on ultrathin sections of the film before and after PCBM doping. For the latter, we removed the PCBM in situ on the TEM grid with hexane to avoid disrupting the polymer network (verified spectroscopically). Hexane is a non-solvent for the polymer. No sample staining or supporting film was used to avoid structural artefacts. The images were collected in the weak defocus regime (−100 nm), where the phase-contrast transfer function is well behaved down to spatial wavelengths of ca . 0.5 nm, to avoid phase artefacts. 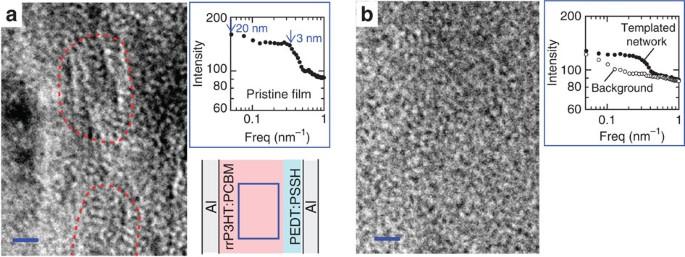Figure 2: High-resolution transmission electron microscopy phase-contrast images of ultrathin polymer sections. (a) Pristine P3HT film and (b) nanotemplated P3HT network film prepared in the same way as devices (Scale bars are 10 nm). The images were collected at 300 keV in the weak defocus regime (−100 nm), without sample staining or supporting film. Approximate semicrystalline domain boundaries were marked inabased on phase coherence as guide to eye. The PCBM nanophase fraction has been extracted with hexane to leave the polymer network inb. The diffractograms were obtained by fast Fourier transform of the images and plotted against spatial frequency. The bottom right panel inashows a schematic of the film configuration and location of the image (blue box). The Al strip suppresses charging and provides stability for extended imaging. The same film configuration was used forb. Figure 2 shows a representative set of images. The cross-section of the pristine P3HT film ( Fig. 2a ) shows the typical coarse texture characteristic of semicrystalline polymers. The diffractogram shows enhanced intensities at 3 nm and 10- to 20 nm spatial wavelengths, which are attributed to the lamellar order of P3HT and its crystalline domain size, respectively [20] . In contrast, the cross-section of the network film gives an ultrafine ‘curly’ texture with no long-range correlation between neighbouring features. Its diffractogram shows the 10- to 20 nm spatial wavelength feature is fully suppressed to the background. Therefore, doping PCBM into the crosslinked P3HT film swells the network and destroys long-range order but not the local interchain stacking order. The observed texture is thus consistent with the proposed ultrafine contiguous polymer network, where network continuity is assured by crosslinking. In contrast, demixed biblend films exhibit a wildly variable texture from the ultrafine to the coarse depending on film-preparation conditions [3] , [9] , [14] . Figure 2: High-resolution transmission electron microscopy phase-contrast images of ultrathin polymer sections. ( a ) Pristine P3HT film and ( b ) nanotemplated P3HT network film prepared in the same way as devices (Scale bars are 10 nm). The images were collected at 300 keV in the weak defocus regime (−100 nm), without sample staining or supporting film. Approximate semicrystalline domain boundaries were marked in a based on phase coherence as guide to eye. The PCBM nanophase fraction has been extracted with hexane to leave the polymer network in b . The diffractograms were obtained by fast Fourier transform of the images and plotted against spatial frequency. The bottom right panel in a shows a schematic of the film configuration and location of the image (blue box). The Al strip suppresses charging and provides stability for extended imaging. The same film configuration was used for b . 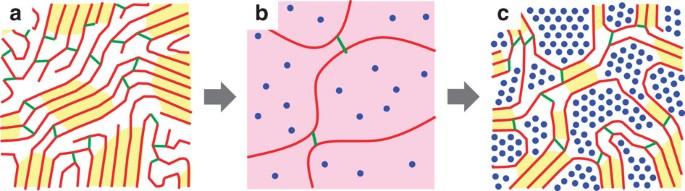Figure 3: A model of the nanotemplating mechanism that produces an ultrafine contiguous polymer network morphology. (a) The polymer (red chains) comprising ordered (yellow) and amorphous domains is lightly crosslinked (green links) to give a swellable network. (b) This network expands in contact with the solvent to allow for incorporation of guest and solvent molecules. (c) As the solvent evaporates, the network contracts, and its morphology becomes nanotemplated by the incorporated guest molecules. The properties of the resultant morphology, such as phase length scale, order and connectivity, are determined more by the crosslink density than solvent or drying conditions or the film thickness. Full size image The nanotemplating mechanism Figure 3 outlines a simple model of the nanotemplating mechanism that produces the ultrafine contiguous polymer network morphology. First, the P3HT chains are crosslinked just above the gel point through their alkyl side chains ( Fig. 3a ). This may be expected to occur primarily in the amorphous regions. Contact with a good solvent then causes the network to swell and expand to a mesh with length scale determined by ~ ρ −1 , which is of the order of 50 repeat units here ( Fig. 3b ). This provides room for guest incorporation. As the solvent evaporates, the polymer network contracts around the PCBM phase. This appears to be determined by P3HT…P3HT and P3HT…PCBM interactions in the presence of the crosslinks that restricts long-range diffusion but allows local ordering of the chain segments. PCBM has limited solubility in the ordered P3HT stacks [9] , [21] . Annealing this network further improves P3HT order, but cannot cause the usual phase coarsening and breakup. In this way, the conflicting demands on length scales (ultrafine but contiguous) can be built into the morphology, predefined to a large extent by the crosslink density. Figure 3: A model of the nanotemplating mechanism that produces an ultrafine contiguous polymer network morphology. ( a ) The polymer (red chains) comprising ordered (yellow) and amorphous domains is lightly crosslinked (green links) to give a swellable network. ( b ) This network expands in contact with the solvent to allow for incorporation of guest and solvent molecules. ( c ) As the solvent evaporates, the network contracts, and its morphology becomes nanotemplated by the incorporated guest molecules. The properties of the resultant morphology, such as phase length scale, order and connectivity, are determined more by the crosslink density than solvent or drying conditions or the film thickness. Full size image Ion-sputtered X-ray photoemission spectroscopy shows that these crosslinked P3HT network: PCBM films exhibit a markedly smaller P3HT surface enrichment and PCBM subsurface enrichment than the usual demixed biblend films. Both the amplitude and width of the composition wave are suppressed ( Supplementary Fig. S2 and Supplementary Discussion ). Thus, the usual formation of an unfavourable P3HT-rich surface layer upon annealing of the biblend films [9] , [22] is greatly attenuated. This is yet another benefit of the crosslinked network. Thus, these films can advantageously produce high PCE ( vide infra ) even without post-cathode annealling [4] , [9] . The PCE landscape Crosslinked P3HT network: PCBM solar cells were fabricated with poly(3,4-ethylenedioxythiophene):poly(styrenesulphonic acid) (PEDT:PSSH) as hole collector and Ca/Al as electron collector. 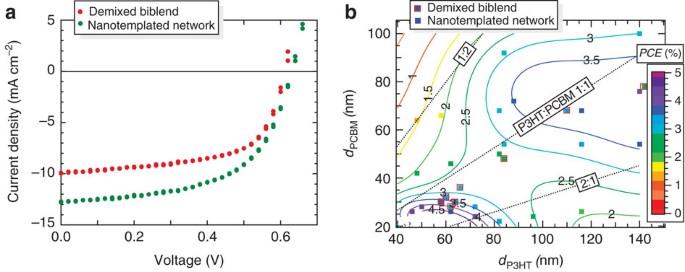Figure 4: Photovoltaic characteristics of glass/130 nm ITO/50 nm PEDT:PSSH/P3HT:PCBM/Ca solar cells under an equivalent solar irradiation of 1.2 sun. (a) Current–voltage characteristics of an optimized demixed biblend device and a crosslinked polymer network: fullerene device:d=85 nm;dPCBM/dP3HT=0.56. (b) Power conversion efficiency landscape, PCE versus (dP3HT,dPCBM), wherediis the effective component thickness. Cell efficiencies are given by colour-coded symbols. Those of demixed biblend cells have a red border. Precision is ±0.15% (absolute). Data are spectral-mismatch corrected. The network cell data are interpolated using a two-dimensional, multi-Gaussian surface (goodness-of-fit,χ2≈1.5). The biblend data fall below this surface by 20 (±10) %. The 1:1 w/w P3HT:PCBM ratio is given by the linedPCBM=0.65 *dP3HT. Other composition lines are as indicated. Figure 4a shows the current–voltage characteristic of such a solar cell compared with one fabricated with the usual demixed biblend film. The cells have the same 1:1 weight-to-weight (w/w) P3HT:PCBM ratio (that is, d PCBM / d P3HT =0.65) and film thickness (85 nm), and were measured together under 1.2 sun illumination (this power setting was chosen for historical reasons; reported PCE is normalised and spectral-mismatch corrected). The network cell shows a markedly higher short-circuit current density j sc (12.6 versus 9.9 mA cm −2 ), a marginally higher open-circuit voltage V oc (0.63 versus 0.61 V), and a similar fill factor FF (0.63), as the biblend cell. As a result, this network cell gives a PCE of 4.2%, which is 30% higher than the biblend cell of 3.2% (averaged over 8 devices). As the devices were measured in the same simulator, they are not subjected to calibration uncertainties. Figure 4: Photovoltaic characteristics of glass/130 nm ITO/50 nm PEDT:PSSH/P3HT:PCBM/Ca solar cells under an equivalent solar irradiation of 1.2 sun. ( a ) Current–voltage characteristics of an optimized demixed biblend device and a crosslinked polymer network: fullerene device: d =85 nm; d PCBM / d P3HT =0.56. ( b ) Power conversion efficiency landscape, PCE versus ( d P3HT , d PCBM ), where d i is the effective component thickness. Cell efficiencies are given by colour-coded symbols. Those of demixed biblend cells have a red border. Precision is ±0.15% (absolute). Data are spectral-mismatch corrected. The network cell data are interpolated using a two-dimensional, multi-Gaussian surface (goodness-of-fit, χ 2 ≈1.5). The biblend data fall below this surface by 20 (±10) %. The 1:1 w/w P3HT:PCBM ratio is given by the line d PCBM =0.65 * d P3HT . Other composition lines are as indicated. Full size image To understand the origin of this improvement, we fabricated solar cells over a wider composition space to map out the PCE landscape, that is, the dependence of PCE on ( d P3HT , d PCBM ). We used a simple combinatorial approach to dope predetermined amounts of PCBM into various thicknesses of crosslinked P3HT films. Figure 4b gives the measured PCE landscape as a colour-coded image plot. The PCE data for the network cells are shown without border. These are then fitted with a two-dimensional, multi-Gaussian model to interpolate the PCE surface contours as guide to the eye. Biblend cells were also fabricated for comparison, along the 1:1 w/w P3HT:PCBM composition ratio, which is known to be nearly optimal [21] . Their PCE data are colour-coded in the same way, but distinguished by a red border. The PCE landscape reveals a high-efficiency composition ridge that is oriented near, but not exactly on, the 1:1 composition line. This ridge is characterized by a strong oscillation in the film-thickness direction with rapid fall off to both sides. The first and second PCE peaks on this ridge are located at ( d P3HT , d PCBM )=(50 nm, 25 nm) and PCE=4.5%, and ( d P3HT , d PCBM )=(125 nm, 75 nm) and PCE=4.0%, respectively, separated by a relative saddle dip of 30%. These two peaks have similar PCEs. The PCE oscillation is widely anticipated from the oscillation of power absorbed within the photoactive layer due to optical interference [8] , [23] , [24] , [25] , [26] . Because of this optical interference effect, devices need to be compared at matched ( d P3HT , d PCBM ) to determine whether there has been a relative improvement. This can be done using the interpolated PCE surface. The PCE of the biblend cell clearly falls below the PCE of the network cell at matched ( d P3HT , d PCBM ) by 10–30%. The biblend cells here show the best PCE of 3.4% in the vicinity of the first PCE peak. This is similar to the best results that have been widely reproduced (3.0–3.6%) [4] , [5] , [8] , [9] , [14] , [21] , although 4–5% have also been reported [27] , [28] . The general improvement in PCE here of ca . 20% in the network cells is remarkable, since the demixed biblend films already exhibit rather good internal quantum efficiencies. Achieving a high second PCE peak is beneficial for manufacturing because this peak is broad and has better defect tolerance. The one-dimensional photonic structure effect revisited The availability of a high quality PCE landscape prompts a re-evaluation of the optical interference effect. We used a standard transfer matrix formalism [29] to compute the photon flux absorbed, Φ ph , in the photoactive layer for the schematic cell structure shown in Fig. 5a , across the entire composition space. The reflective electrode causes optical field nodes and antinodes to emerge within the cell, as has previously been well known in organic light-emitting diodes [30] . This systematically alters the efficiency of the cell in absorbing light, which needs to be determined. The complex dielectric functions of all the layers were known or measured, together with the spectral irradiance of the solar simulator and the composition dependence of for the photoactive layer. 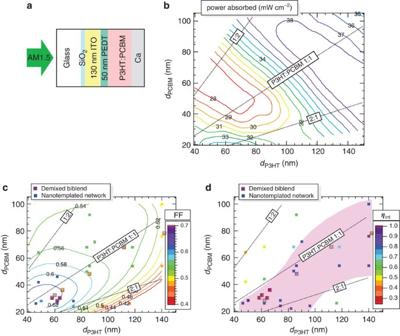Figure 5: The power absorbed, fill factor and internal quantum efficiency landscapes for nanotemplated network solar cells. (a) Optical model of the P3HT:PCBM solar cell to compute the power absorbedPabsin the photoactive layer. (b) Computed composition dependence ofPabsfor the experimental solar irradiance (1.2 sun). (c) Measured composition dependence of the fill factor FF. The network cell data are interpolated with a polynomial surface (goodness-of-fit,χ2≈1.4). (d) Composition dependence of the internal photon-to-electron conversion quantum efficiencyηintat zero bias. The shaded magenta region is a guide to the eye whereηint≈0.85, obtained from the modelled PCE and FF surfaces together with the computedΦph. Figure 5: The power absorbed, fill factor and internal quantum efficiency landscapes for nanotemplated network solar cells. ( a ) Optical model of the P3HT:PCBM solar cell to compute the power absorbed P abs in the photoactive layer. ( b ) Computed composition dependence of P abs for the experimental solar irradiance (1.2 sun). ( c ) Measured composition dependence of the fill factor FF. The network cell data are interpolated with a polynomial surface (goodness-of-fit, χ 2 ≈1.4). ( d ) Composition dependence of the internal photon-to-electron conversion quantum efficiency η int at zero bias. The shaded magenta region is a guide to the eye where η int ≈0.85, obtained from the modelled PCE and FF surfaces together with the computed Φ ph . Full size image Figure 5b shows the computed dependence of power absorbed P abs on ( d P3HT , d PCBM ) at the spectral irradiance used in the experiments. The plot clearly shows a strong diagonal oscillation along the photoactive layer thickness direction and a weaker compositional dependence at fixed thicknesses, particularly for the thicker films. The first and second absorption peaks are located at ( d P3HT , d PCBM )=(60 nm, 20 nm), 34 mW cm −2 , and (130 nm, 70 nm), 38 mW cm −2 , respectively. These correspond to the emergence, respectively, of one and two optical field antinodes in the photoactive layer. The second peak is within a few per cent of the theoretical maximum in the photoactive layer, after taking into account reflection and parasitic ITO and PEDT:PSSH losses. Despite the small d of 80 nm at the first optimum, the P abs is only ca . 12% lower than the second optimum at 200 nm. This is because of strong optical field enhancement in the centre of the thin film. Furthermore, the computed plot explains the curious displacement of the first optimum towards the 2:1 P3HT-rich composition line. This is because the power absorbed scales strongly with absorptivity in this regime. It is evident that the PCE landscape bears the signatures of the P abs surface. This provides first unambiguous evidence for the role of optical interference in determining the PCE of organic solar cells, through its influence on absorption in the photoactive layer. The FF landscape To probe the influence of controlled DA morphology in the network cells on the shape of their current-voltage characteristics, we plotted FF as a function of ( d P3HT , d PCBM ) in Fig. 5c . We found the FF decreases gently with increasing d but more strongly with increasing off-compositions from the 1:1 line. The gradual decrease with d arises from the space-charge voltage penalty that sets in when the carrier extraction distance becomes long [31] , together with a possible (weak) field dependence of the charge-separation step [32] . The strong composition-ratio dependence on composition, in particular its pronounced asymmetry, on the other hand, can be attributed to the underlying phase connectivity of the DA morphology. As the film composition becomes P3HT rich, the PCBM nanophase eventually becomes poorly connected. This causes the effective electron mobility to drop and the photocurrent to become space-charge limited. However, as the film composition becomes PCBM rich, the converse does not occur as readily, because the crosslinked P3HT network ensures built-in phase continuity for the hole carriers. This FF landscape thus reveals an interesting morphology aspect of these nanotemplated crosslinked networks. Detailed modelling of the current–voltage curves along the high-efficiency ridge reveals that the effective hole mobility is ca. 2 × 10 −4 cm 2 V −1 s −1 , largely independent of film thickness. This shows that the morphology is indeed well regulated (Liu et al ., unpublished). The internal quantum efficiency landscape Finally we analyse the landscape of the internal quantum efficiency η int , that is, electron collected per photon absorbed, of these cells at short-circuit to reveal another feature of the DA morphology. The η int is a measure of the photocurrent generation quantum yield of the photoactive layer. This can be phenomenologically written as , where η gen is the photo-carrier generation efficiency, that is, fraction of excitons dissociated to carrier pairs, and η coll is their collection efficiency, that is, the fraction of carrier pairs collected at the electrodes without undergoing recombination. Since both these steps are strongly morphology dependent, η int is a useful proxy to characterize the effectiveness of the DA heterostructure to generate photocurrent. Figure 5d shows the dependence of η int on d P3HT and d PCBM , extracted at zero bias from j sc according to the following formula: , where q is the elementary charge and Φ ph is the computed photon flux absorbed (cm −2 s −1 ) in the photoactive layer. The η int landscape thus reveals a broad high-efficiency ridge (shaded magenta to guide the eye) that is disposed between the 1:1 and 2:1 P3HT:PCBM composition lines. However, unlike the PCE ridge, this is substantially free from oscillations. The η int is 0.85 over most of the shaded region, rising marginally to 0.9 in the vicinity of the first PCE peak, but falling off strongly to its sides. Thus, the roll-off in the PCE for strongly off-optimal compositions is due to the sharp decline in η int . This is caused by the very imbalanced donor and acceptor phase ratio. Hence, it is clear that the overall PCE surface can be separated into a photonic structure contribution and a DA morphology contribution. The high η int values found across a wide swathe of ( d P3HT , d PCBM ) space is noteworthy. It shows that both photo-carrier generation and collection efficiencies can approach near unity over a wider composition space than previously thought possible. Although high η int values can also be reached in demixed biblend cells, for example, in the vicinity of the first PCE peak ( η int ~0.8), this drops quickly with d to ca . 0.6 in the vicinity of the second peak. We attribute this to a progressive drift in the DA morphology of thicker demixed films [13] . Previous current–voltage modelling [33] and transient spectroscopy [32] , [34] have shown that the primary loss mechanisms in these films are geminate and non-geminate recombinations, each accounting for ca . 10% losses in thin films. The even higher efficiencies of the nanotemplated network cells reached here show these mechanisms can be further suppressed. Although the above results have been established using CB as the processing solvent, we note that both the optical characteristics of the doped polymer network and the electrical characteristics of their cells are rather insensitive to the choice of processing solvent. For example, this could be changed to chloroform or 1,2-dichlorobenzene to cover two decades in solvent volatility and film drying time without causing any significant change to the characteristics of the final films, according to electronic spectroscopy ( Supplementary Fig. S3 ) and the solar cell characteristics ( Supplementary Fig. S4 ; see also Supplementary Discussion ). This is in marked contrast to the well-known sensitivity of the properties of spin-cast biblend films. The novelty of this work lies in the demonstration that high η int (and PCE) can be achieved consistently across a wide swathe of ( d P3HT , d PCBM ) space using a simple method of PCBM acceptor doping into a lightly crosslinked P3HT donor polymer matrix, in which phase connectivity and length scale are preset by the crosslink density. As a result, the desired ultrafine morphology can be produced with rather weak sensitivity to film thickness, solvent processing and annealing conditions. This methodology can thus be consistently implemented over large film areas and thicknesses, and be potentially manufactured on scale. More fundamentally, this work reveals an approach to decouple the DA morphology from electronic structure. This is exciting because it allows separate control and hence optimization of these two vital aspects. This approach when used with state-of-the-art materials will likely underpin further advances. Finally, it appears that not only molecular acceptors but monomers, oligomers and nanorods may also be infiltrated into the crosslinked networks. This will greatly enhance the versatility of these networks, not only for solar cell but also other applications that require a controlled ultrafine morphology, perhaps in energy storage. Materials P3HT (Sigma Aldrich, >98% head-to-tail regioregularity, MW 30–60 kDa) and PCBM (Nano-C) were used as received. The s -FPA crosslinker was synthesized in-house following established procedures [16] . Photocrosslinking was performed in a glove box ( p O 2 ; p H 2 O<1 ppm) with a 254-nm-wavelength DUV exposure at a dose of ca . 300 mJ cm –2 from an 8-W low-pressure Hg lamp. Device fabrication and characterization Solar cell devices were fabricated on ITO-coated glass substrates. The substrates were first cleaned with an SC-1 recipe. PEDT:PSSH (1:16 w/w; reformulated Baytron P; Leverkussen) films of 50 nm thickness were spin-cast and annealed at 120 °C in the glove box to remove sorbed moisture. The P3HT:PCBM films were then formed in the glove box, either by spin-casting of biblend mixtures (18–24 mg ml −1 ) or by PCBM doping of crosslinked P3HT films. All photoactive layers were processed from CB. To fabricate the crosslinked polymer network: fullerene devices, P3HT was dissolved in CB (10–20 mg ml −1 ) with 3 weight% ethylene bis(4-azido-2,3,5-trifluoro-6-isopropylbenzoate (referred to P3HT=100%) as the crosslinker additive. The films were spin-cast and crosslinked by DUV exposure, and then washed with CB twice on the spinner. PCBM was dissolved in CB (8–30 mg ml −1 ) and spun at different speeds onto the crosslinked P3HT films. The thicknesses of the photoactive layers lie between 80 and 220 nm for both biblend and doped network films. All devices were then annealed in the glove box at 140 °C for 10 min (hotplate), before evaporating a 30-nm-thick Ca electrode capped with 120-nm-thick Al at a base pressure of better than 1 × 10 −6 Torr. Eight devices (4.3 mm 2 each) were prepared and measured on each substrate. The density of the P3HT nanophase in the photoactive layer was assumed to be 1.1 g cm −3 , on the basis of its known crystalline density (1.16 g cm −3 , ref. 35 ). The density of the PCBM nanophase was assumed to be 1.7 g cm −3 , on the basis of the known crystalline densities of the 1:0.5 adduct of the PCBM:CB complex (1.65 g cm −3 ) and the 1:1 adduct of the PCBM:1,2-dichlorobenzene complex (1.67 g cm −3 , ref. 36 ) which set a lower bound due to the incorporation of solvent molecules. The ratio of these densities is consistent with our measurements of d P3HT and d PCBM . Current–voltage characteristics were measured on a Keithley 4200 semiconductor characterization system. The cells were illuminated with the simulated AM1.5 spectral output (at 1.2 sun) of a home-built solar simulator with Xe arc lamp corrected with an AM1.5G filter. This simulator was cross-calibrated with a commercial-class ABA solar simulator (Oriel Sol2A), which in turn was cross-checked by calibration services at Solar Energy Research Institute of Singapore. Spectral-mismatch correction was applied to the reported results. Optical modelling The standard optical transfer matrix method was used to model the optical absorption of the solar cells. The complex dielectric functions of all the layers were either known or measured in this work over the 400 to 650 nm wavelength range. The dielectric functions of P3HT:PCBM layer were measured by variable-angle spectroscopic ellipsometry on annealed biblend films, with weight ratios 1:2, 1:1 and 2:1, and then interpolated by Bruggeman effective medium approximation to obtain the compositional dependence at 5 nm wavelength steps and on a 10-nm ( d P3HT , d PCBM ) grid. The fractional absorption of the photoactive layer was computed from the difference in Poynting vectors. The integrated absorbed power and photon flux for the experimental solar simulator were then computed at 2 nm steps using the measured incident spectral irradiance taking care of reflection at the air/glass interface. How to cite this article: Liu, B. et al . High internal quantum efficiency in fullerene solar cells based on crosslinked polymer donor networks. Nat. Commun. 3:1321 doi: 10.1038/ncomms2211 (2012)